Draft genome sequence and genetic transformation of the oleaginous algaNannochloropsis gaditana The potential use of algae in biofuels applications is receiving significant attention. However, none of the current algal model species are competitive production strains. Here we present a draft genome sequence and a genetic transformation method for the marine microalga Nannochloropsis gaditana CCMP526. We show that N. gaditana has highly favourable lipid yields, and is a promising production organism. The genome assembly includes nuclear (~29 Mb) and organellar genomes, and contains 9,052 gene models. We define the genes required for glycerolipid biogenesis and detail the differential regulation of genes during nitrogen-limited lipid biosynthesis. Phylogenomic analysis identifies genetic attributes of this organism, including unique stramenopile photosynthesis genes and gene expansions that may explain the distinguishing photoautotrophic phenotypes observed. The availability of a genome sequence and transformation methods will facilitate investigations into N. gaditana lipid biosynthesis and permit genetic engineering strategies to further improve this naturally productive alga. In recent years, a detailed understanding of the many biosynthetic pathways that can be used for the production of biofuel feedstocks or higher value bioproducts has emerged, and novel pathways for the production of specific bioenergy carriers are continuously being discovered in a variety of organisms [1] , [2] , [3] , [4] . These advances, in combination with the development of reliable genetic transformation protocols for photosynthetic organisms with high innate biomass accumulation rates will enable the engineering of improved strains that not only have high production rates but also produce tailored precursors, or even finished products of biotechnological interest [2] , [5] , [6] , [7] . Several species of Nannochloropsis have attracted sustained interest from algal biofuels researchers owing to their high photoautotrophic biomass accumulation rates, high lipid content [8] , [9] , [10] , [11] , [12] , and their successful cultivation at large scale using natural sunlight in either open ponds or enclosed systems by companies such as Solix Biofuels, Aurora Algae, Seambiotic, Hairong Electric Company/Seambiotic and Proviron. Further improvements in strain productivity have been hampered by the lack of a genetically tractable model system for these highly productive oleaginous algae. Currently, the most developed algal model species are the green alga Chlamydomonas reinhardtii and the diatom Phaeodactylum tricornutum , both of which have genome sequences and established transformation methods [13] , [14] , [15] , [16] , [17] , [18] . Genetic engineering approaches have been successfully used to improve biofuel phenotypes in both of these organisms [19] , [20] , [21] , [22] ; unfortunately, neither of these algae is a natively exceptional producer of biomass or lipids, and, as such, extensive genetic modifications will be needed before their use in biofuel applications. An alternative alga that has inherently desirable biomass production characteristics and has been successfully cultivated outdoors at commercial scale is Nannochloropsis gaditana , a stramenopile alga in the Eustigmatophyceae, which is oleaginous and stores relatively large amounts of lipid, in the form of triacylglycerides (TAG), even during logarithmic growth. Various strains of Nannochloropsis have been investigated for their biomass and lipid production characteristics, and several isolates have been grown for aquaculture purposes. N. salina, N. oculata and N. gaditana have received the most attention because of their exceptional lipid production characteristics [9] , [23] , [24] . N. gaditana has high photoautotrophic biomass and lipid production rates and can grow to high densities (>10 g l −1 ) while tolerating a wide range of conditions with regards to pH, temperature and salinity. N. gaditana is therefore a good candidate for development into a model organism for algal biofuel production, and the availability of a genome sequence and reliable transformation protocols are required advances in this direction. In addition, there are reports that homologous recombination is tractable in the eustigmatophyte Nannochloropsis W2J3B [25] , [26] . In this study, to transform a natively robust and oleaginous alga into a model system for biofuel production, we sequenced the genome and developed a genetic transformation method for N. gaditana CCMP526. We also investigated the N. gaditana lipid metabolic pathways on the genome and transcriptome levels, quantifying gene transcript levels during a relatively low lipid production stage, (logarithmic growth), and a high lipid production stage, (stationary phase) after nitrate depletion. Finally, we conducted comparative phylogenomic analyses among other algal lineages to determine genes unique to N. gaditana and to identify sets of conserved proteins across photosynthetic stramenopiles. The genome sequence, its analysis, and the development of genetic transformation in N. gaditana are important first steps in improving this industrially proven, oleaginous algal for biofuel production. High lipid yields from high-density cultures of N. gaditana N. gaditana is a robust producer of both biomass and lipids under a wide array of culture conditions, including minimal f/2 seawater medium and artificial seawater (10–120% seawater salinity, pH 7–10) supplemented with nitrate, phosphate and CO 2 . 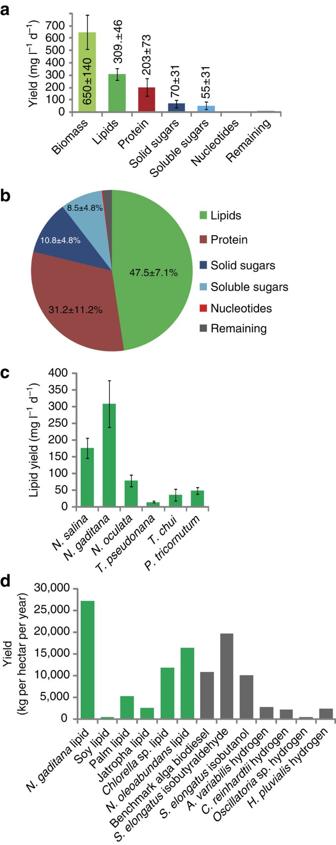Figure 1: Biomass production byN. gaditana. (a)N. gaditanaproduction of biomass, lipids, protein and sugars quantified during continuous growth over a period of 3 months in 50% salinity seawater medium supplemented with nitrate, phosphate and CO2with continuous 1,000 μE light. Every week, half of the culture was collected and replaced with fresh medium. Inset values show the yield in mg l−1per day. Values are from 12 measurements and error bars show the standard deviation. (b) Chart illustrating collected biomass compositions, the majority of which consists of lipids even under nutrient replete conditions. Inset values show percentage of total biomass. (c) Comparison ofN. gaditanalipid production rates with other algae examined in this work. Values are from at least three separate experiments and error bars show the standard deviation. (d) Comparison ofN. gaditanalarge-scale production rates with other biofuel production platforms. Bars in green indicate our estimations; bars in grey indicate estimations by Atsumiet al.30The values forN. gaditanahave been extrapolated from 1 l cultures and adjusted for our observed productivity in 12 h/12 h light/dark cycles. TheS. elongatusproduction values are for 24 h light and would presumably be lower in 12 h/12 h light/dark cycles. The yields from N. gaditana cultures grown in f/2 medium at 50% seawater salinity are shown in Figure 1a,b . Yields of 0.65 g l −1 d −1 biomass and 0.31 g l −1 d −1 total lipids were achieved over a period of 3 months in 1 l Roux Flasks sparged with air/2% CO 2 , when half the cultures were exchanged for fresh medium every week. Lipid body accumulation can be triggered/enhanced in most algae by nitrogen deprivation or other stress conditions [27] , and the high lipid content (47.5%) in actively growing cultures of N. gaditana is likely facilitated by the rapid depletion of nitrate in dense cultures (3–8 g l −1 ) during growth. Optimal lipid yields were obtained with a starting culture density of ~3.6 g l −1 . It is likely that lack of light penetration due to self-shading is the main limiting factor for cultures at higher starting densities. Low-density cultures (<0.5 g l −1 ) can be growth inhibited by high light (>200 μE) but the higher density cultures have good production between 1,000 μE and 2,000 μE. For medium to high-density cultures (3–10 g l −1 ), no substantial increase in productivity is observed on increasing the light from 1,000 μE to 2,000 μE, supporting the hypothesis that self shading becomes the limiting factor at these densities. The laboratory productivity numbers have been extrapolated to calculate potential lipid yields in comparison with other algae ( Fig. 1c ) and to other biofuel production platforms ( Fig. 1d ). In Figure 1d , the green bars indicate our extrapolations based on data from Chisti et al . [28] and Chen et al . [29] , whereas grey bars indicate estimations originally provided by Atsumi et al . [30] It is important to note that some of the values represent actual production yields from large-scale cultivation (Soy, Palm) [28] , [31] , whereas other values are extrapolated from small scale cultures with 24 h light ( Synechococcus elongatus Isobutyraldehyde and Isobutanol). The N. gaditana lipid production yields have been derived from small scale cultures with 12 h light/12 h dark cycles and therefore provide a more realistic estimation relative to S. elongatus . Robust lipid yields from Nannochloropsis scale from 25 ml cultures to 8 l cultures under laboratory conditions, to 10-hectare outdoor ponds where it is grown on a commercial scale (Hairong Electric Company and Seambiotic). The high lipid content of N. gaditana cells is apparent on fluorescent labelling of algal triglycerides with the lipophilic dye, BODIPY. Actively growing cells have a constitutive lipid droplet that expands within cells in stationary phase or during nitrogen deprivation ( Supplementary Fig. S1a,b respectively). The large majority of lipids in N. gaditana are composed of palmitic and palmitoleic acid with a minor content of myristic and oleic acid ( Supplementary Fig. S1c ), resulting in a relatively simple fatty acid profile, and these fatty acids can be used for the production of biodiesel or biopetrol. Figure 1: Biomass production by N. gaditana . ( a ) N. gaditana production of biomass, lipids, protein and sugars quantified during continuous growth over a period of 3 months in 50% salinity seawater medium supplemented with nitrate, phosphate and CO 2 with continuous 1,000 μE light. Every week, half of the culture was collected and replaced with fresh medium. Inset values show the yield in mg l −1 per day. Values are from 12 measurements and error bars show the standard deviation. ( b ) Chart illustrating collected biomass compositions, the majority of which consists of lipids even under nutrient replete conditions. Inset values show percentage of total biomass. ( c ) Comparison of N. gaditana lipid production rates with other algae examined in this work. Values are from at least three separate experiments and error bars show the standard deviation. ( d ) Comparison of N. gaditana large-scale production rates with other biofuel production platforms. Bars in green indicate our estimations; bars in grey indicate estimations by Atsumi et al . 30 The values for N. gaditana have been extrapolated from 1 l cultures and adjusted for our observed productivity in 12 h/12 h light/dark cycles. The S. elongatus production values are for 24 h light and would presumably be lower in 12 h/12 h light/dark cycles. Full size image Sequencing and assembly DNA sequencing reads obtained, using both Roche and Illumina (including both unpaired and LIPES protocols) technologies, were trimmed for quality, and then assembled separately. These assemblies were merged, followed by removal of scaffolds of bacterial contaminant(s), producing a genome assembly of 2,087 scaffolds, with an N50 of 257 and an L50 of 37,693 nucleotides (nts) ( Table 1 ). There are 35 scaffolds longer than 100 kb, a total of 561 longer than 20 kb, and a total of 1,447 that are longer than 2 kb. Table 1 also includes statistics on the contigs before assembly into the final scaffolds. Table 1 N. gaditana genome statistics. Full size table In addition to the nuclear genome, the plastid and mitochondrial genomes were also sequenced, assembled and annotated ( Supplementary Figs S2 and S3 ). Relative to the organellar genomes of P. tricornutum and Thalassiosira pseudonana , significant conservation of gene content and gene organization was observed, with some notable exceptions [32] . See Supplementary Note 1 and Supplementary Table S1 for a detailed description. RNA was isolated from a variety of culturing conditions and growth phases, converted into complementary DNA (cDNA), then sequenced using the Illumina SIPES protocol, followed by assembly of these reads using the commercial package from CLC Bio (Katrinebjerg) into 37,055 contigs. Genome annotation A variety of methods were used, including ab initio predictions, homology detection, and RNAseq matching to the genome assembly, and then these were reconciled into a single gene set using Maker [33] . Contigs from the transcript assembly that had strong homology support, but were otherwise not part of the Maker gene set, were added to form gene set version 1.1 with 9,052 members ( Table 1 and Supplementary Table S2 ). We identified several functional gene clusters, including a uniquely arranged cluster of four genes involved in hydrogenase function ( HYDA1 , HYDE , HYDF and HYDG ) and a cluster of three genes involved in nitrogen assimilation (nitrate reductase, nitrite reductase, and a nitrate transporter) ( Supplementary Fig. S4 ). Similar clusters of nitrogen assimilation genes can be observed in prasinophytes and C. reinhardtii [34] , [35] . However, despite the presence of other functional clusters, no nitrogen assimilation gene cluster can be observed in the more closely related Ectocarpus siliculosus [36] . An expanded analysis of functional gene clusters can be found in Supplementary Note 2 and Supplementary Table S3 . Comparative genomics N. gaditana is a eustigmatophyte alga that is closely related to the Phaeophyceae (brown algae), with the most closely related organism having a fully sequenced genome being the multicellular brown alga, E. siliculosus ( Fig. 2a ) [36] . Among other species of Nannochloropsis , N. gaditana is most closely related to N. salina ( Fig. 2b ). To identify novel features of the N. gaditana genome, we determined which N. gaditana genes have homologues found in brown algae [36] and the pelagophyte Aureococcus. anophagefferens [37] ), green algae ( Chlorella variabilis NC64A [38] and C. reinhardtii [13] ), red algae ( Cyanidioschyzon merolae [39] ), and diatoms ( T. pseudonana [40] and P. tricornutum [14] ). This analysis confirms the close evolutionary proximity between the Eustigmatophyceae and Phaeophyceae ( Fig. 2c ), and provides us with 2,733 genes that are exclusive to N. gaditana , not found in the other algal genomes queried. This corresponds to 30.2% of the total gene repertoire in N. gaditana , which is similar to the fraction of unique genes found in T. pseudonana [40] , E. siliculosus [36] and P. tricornutum [14] . Comparison of N. gaditana gene models to the non-redundant protein database (BLASTp) yielded top hits from a variety of organisms, the most frequent being stramenopiles ( Fig. 2d ), which was expected on the basis of the phylogeny of N. gaditana . 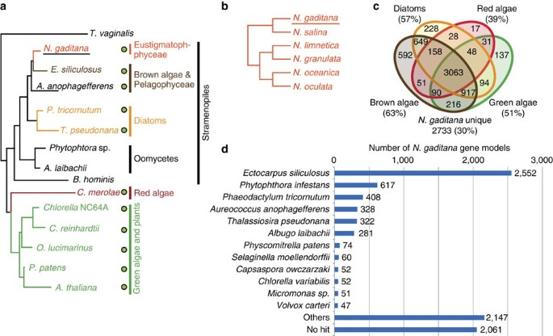Figure 2: Phylogenetic analysis of theN. gaditanagenome. (a) Schematic phylogenetic tree of stramenopiles and photosynthetic algae. The tree is adapted from Eisenreichet al.,43and Tyleret al.60Filled green circles on the right indicate photosynthetic species. (b) The tree indicates the relationship between different strains ofNannochloropsisbased on 18S ribosomal RNA gene sequences. (c) Venn diagram representation of shared/unique genes ofN. gaditanain comparison with brown algae, diatoms, red algae and green algae. (d)N. gaditanagene models were compared with all previously sequenced genomes in the non-redundant protein database using BLASTp. The number of times an organism was the top BLASTp hits (E-value less than 1E-3) of aN. gaditanagene model is indicated. Figure 2: Phylogenetic analysis of the N. gaditana genome. ( a ) Schematic phylogenetic tree of stramenopiles and photosynthetic algae. The tree is adapted from Eisenreich et al ., [43] and Tyler et al . [60] Filled green circles on the right indicate photosynthetic species. ( b ) The tree indicates the relationship between different strains of Nannochloropsis based on 18S ribosomal RNA gene sequences. ( c ) Venn diagram representation of shared/unique genes of N. gaditana in comparison with brown algae, diatoms, red algae and green algae. ( d ) N. gaditana gene models were compared with all previously sequenced genomes in the non-redundant protein database using BLASTp. The number of times an organism was the top BLASTp hits ( E -value less than 1E-3) of a N. gaditana gene model is indicated. Full size image Previous attempts have been made at establishing the minimal essential set of genes needed for photosynthesis, the 'GreenCut' of photosynthetic genes, which is a set of 597 orthologues that are conserved in plant and green algal lineages, but not in non-photosynthetic organisms [13] , [41] . We decided to take advantage of the fact that there are both photosynthetic and non-photosynthetic stramenopiles to generate an analogous set of genes conserved in photosynthetic stramenopiles. To establish this 'StramenopilePhotoCut' of photosynthetic genes, orthologues common to N. gaditana and four photosynthetic stramenopiles ( E. siliculosus, A. anophagefferens, T. pseudonana and P. tricornutum ), but not present in non-photosynthetic stramenopiles ( Phytophtora sojae, Phytophtora ramorum, Phytophtora infestans, Albugo laibachii or Blastocystis hominis ), were selected, resulting in a list of 363 genes. ( Fig. 3a and Supplementary Data 1 ). The majority of these genes have orthologues in the green and red algal lineages and 115 are found in the 'GreenCut2' [41] . However, 39 genes with homologues only found in photosynthetic stramenopiles are present in the genome ( Supplementary Data 1 ). Similar to many genes found in the 'GreenCut', some of the 39 stramenopile-specific 'StramenopilePhotoCut' genes are of completely unknown function, but several of the genes have known domains, including several peptidases/proteases, DNA-binding proteins/transcription factors, and transport proteins, as well as genes that are thought to directly interact with the photosystems ( Fig. 3b ). Because of the high photoautotrophic growth rates exhibited by N. gaditana , we also characterized the complete pathways for synthesis of chlorophyll and accessory pigments ( Supplementary Table S4 ). All expected genes could be identified except for those encoding the mevalonate (MVA) pathway for isopentenyl-pyrophosphate biosynthesis (see the analysis of bioenergy metabolic pathways). 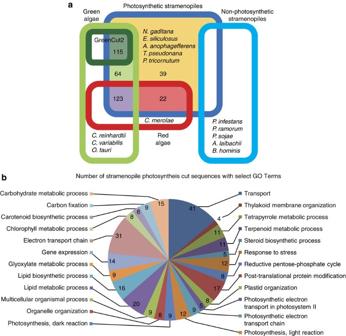Figure 3: Genes conserved in photosynthetic stramenopiles. (a) Euler diagram showing the 363 genes that make up the StramenopilePhotoCut genes common to photosynthetic and absent in non-photosynthetic stramenopiles. Number of genes found in each sector is indicated. The centre yellow sector indicates genes unique for the photosynthetic Stramenopiles (not found in green or red lineages). (b) Chart showing the number of 'StramenopilePhotoCut' genes with select GO terms. 'StramenopilePhotoCut' genes with no GO terms are not indicated. Figure 3: Genes conserved in photosynthetic stramenopiles. ( a ) Euler diagram showing the 363 genes that make up the StramenopilePhotoCut genes common to photosynthetic and absent in non-photosynthetic stramenopiles. Number of genes found in each sector is indicated. The centre yellow sector indicates genes unique for the photosynthetic Stramenopiles (not found in green or red lineages). ( b ) Chart showing the number of 'StramenopilePhotoCut' genes with select GO terms. 'StramenopilePhotoCut' genes with no GO terms are not indicated. Full size image Bioenergy metabolic pathways To investigate metabolic pathways of interest for biofuel production, functional annotations were assigned to N. gaditana gene models. Gene ontology terms (GO-terms) were assigned to 3,838 gene models, from which 2,766 genes were identified as performing enzyme-catalysed reactions representing 700 unique EC numbers that were in turn used to populate metabolic pathway maps ( Fig. 4 ). Some of the most frequent GO-terms, aside from housekeeping functions, are terms involved in auxin biosynthesis, photosynthesis, and lipid biosynthesis ( Supplementary Fig. S5 ). Because of the exemplary lipid production by N. gaditana cultures, we focused on characterizing lipid metabolic pathway genes, including those involved in fatty acid biosynthesis, TAG assembly and lipid activation/degradation ( Supplementary Table S5 ). BLASTp was used to identify homologues of the N. gaditana lipid metabolic genes in red/green/brown algae and diatoms. Comparison of the number of genes in each step of the lipid metabolic pathways suggests that N. gaditana has an expanded repertoire of genes involved in both TAG assembly and lipid degradation, including glycerol 3-phosphate dehydrogenase, glycerol 3-phosphate acyltransferase, diacylglycerol acyltransferase, long-chain acyl-CoA ligase and acyl-CoA oxidase ( Fig. 5 and Supplementary Table S6 ). This increased number of lipid metabolic pathway genes is probably significant considering that N. gaditana has fewer total genes than all other algae used for this comparison, with the exception of C. merolae . To further examine the expansion of gene families in N. gaditana , we compared the prevalence of GO-terms with P. tricornutum and C. reinhardtii using the Fisher's exact test. A selected list of over- and under-represented terms is shown in Supplementary Table S7 . This analysis confirms the overrepresentation of the GO-term for acyl-carrier protein biosynthetic processes and also indicates the expansion of several other gene families that may be of importance for the biomass production phenotype of N. gaditana. These include genes involved in auxin biosynthetic processes, carbon utilization, response to stress (including chemical, temperature and salt), and pyruvate metabolic processes. See Supplementary Note 3 for a more detailed analysis of these gene expansions/reductions. 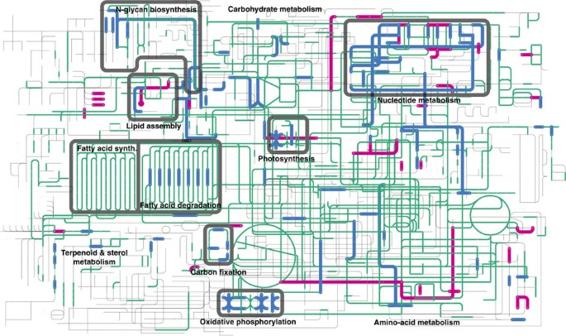Figure 4:N. gaditanametabolic pathway map. Light grey background traces indicate KEGG pathways not encoded by theN. gaditanagenome. KEGG pathways in green, magenta or blue are present in theN. gaditanagenome. Genes that are up- or down-regulated during nitrogen deprivation are labelled in magenta and blue, respectively. Figure 4: N. gaditana metabolic pathway map. Light grey background traces indicate KEGG pathways not encoded by the N. gaditana genome. KEGG pathways in green, magenta or blue are present in the N. gaditana genome. Genes that are up- or down-regulated during nitrogen deprivation are labelled in magenta and blue, respectively. 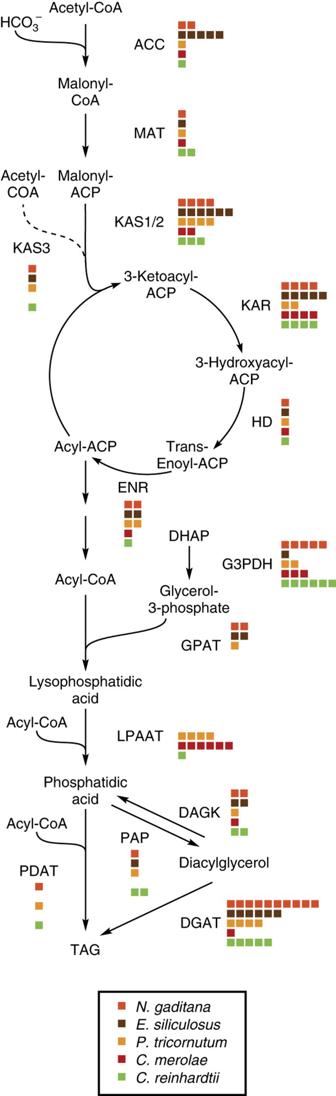Figure 5: Comparison of TAG biosynthetic pathway genes. Number of gene homologues in the TAG biosynthetic pathways inN. gaditanaas compared with a brown alga (E. siliculosus), a diatom (P. tricornutum), a red alga (C. merolae) and a green alga (C. reinhardtii). For each reaction, coloured squares denote the number of homologous genes inN. gaditana(pink),E. siliculosus(brown),P. tricornutum(orange),C. merolae(red),C. reinhardtii(green). Full size image Figure 5: Comparison of TAG biosynthetic pathway genes. Number of gene homologues in the TAG biosynthetic pathways in N. gaditana as compared with a brown alga ( E. siliculosus ), a diatom ( P. tricornutum ), a red alga ( C. merolae ) and a green alga ( C. reinhardtii ). For each reaction, coloured squares denote the number of homologous genes in N. gaditana (pink), E. siliculosus (brown), P. tricornutum (orange), C. merolae (red), C. reinhardtii (green). Full size image To assist in the identification of genes and to improve metabolic pathway maps of N. gaditana , we sequenced the transcriptome (RNAseq) under a variety of physiological conditions. Additionally, transcriptome sequencing was conducted during logarithmic growth (low lipid production) and during stationary phase due to nitrate deprivation (high lipid production) to discover how transcriptional changes in N. gaditana modulate increased metabolic flux into lipid biosynthesis during nutrient deprivation. Genes that are most strongly regulated during these different conditions are shown in Supplementary Data 2 . Similar to the findings in C. reinhardtii [42] , many of the genes that are most strongly upregulated during nitrogen deprivation are genes involved in nitrogen assimilation and protein degradation/recycling, whereas many of the most downregulated genes are involved in photosynthesis. In addition, we annotated the most highly regulated pathways on the metabolic pathway map ( Fig. 4 ). This map highlights the decreased expression of genes involved in photosynthesis, carbon fixation, and oxidative phosphorylation that would be expected during stationary phase owing to nutrient deprivation. Surprisingly, few genes that are directly involved in lipid biosynthesis are transcriptionally upregulated to a significant extent. Because N. gaditana constitutively produces TAG even during logarithmic growth, a possible explanation for this low amount of differential transcript accumulation is that the lipid production machinery may already be abundant within the cell, and existing levels can manage increased metabolic flux. In support of this hypothesis, we found that genes assigned with the GO-term for post-transcriptional regulation of gene expression were overrepresented in N. gaditana in comparison with P. tricornutum and C. reinhardtii , whereas the GO-term for transcription factors was underrepresented ( Supplementary Table S7 ). Interestingly, genes involved in gluconeogenesis (fructose-1,6-bisphosphatase, fructose-1,6-bisphosphate aldolase and phosphoglycerate kinase) are downregulated, which could help direct carbon flux away from carbohydrate biosynthesis into lipid biosynthesis. To determine the exact mechanisms of lipid accumulation during nutrient deprivation, further transcriptomic, proteomic and metabolomic investigations are needed. Other pathways that are of interest for bioenergy applications are the two isoprenoid biosynthesis pathways, the mevalonate and the non-mevalonate pathways (DXP). Ancestral eukaryotes generally have only the MVA pathway although many photosynthetic organisms have acquired the DXP pathway, most probably through a cyanobacterial endosymbiont or secondarily through a red algal symbiont [43] . Interestingly, most higher plants retained both the MVA and DXP pathways, whereas the green and red algae (for example, C. reinhardtii, Ostreococcus lucimarinus, C. merolae ) have kept only the more recently acquired DXP pathway and eliminated the more ancestral MVA pathway. Similarly, N. gaditana and A. anophagefferens have only the DXP pathway ( Supplementary Fig. S6 and Supplementary Table S4 ), whereas other stramenopiles in the case of diatoms and brown algae ( P. tricornutum, T. pseudonana, Ectocarpus siliculosus ) have kept both the MVA and DXP pathways. Parasitic chromalveolates, including stramenopiles, seem to differ in their isoprenoid biosynthesis capacity depending on whether they have kept at least a remnant plastid. Both P. marinus (has a functional plastid) and P. falciparum (has a remnant plastid) have kept the DXP pathway, whereas P. sojae, P. ramorum and A. laibachii (no plastid) have lost both the MVA and DXP pathways. Carbon-concentrating mechanisms Simple mechanisms for carbon concentration and carbon assimilation have been described in many algae [44] . These mechanisms typically rely on carbonic anhydrases, which catalyse the reversible conversion of CO 2 to bicarbonate (HCO 3 − ). The physiological function of a carbonic anhydrase is dictated by its compartmentalization. Bicarbonate cannot passively cross membranes and has to either be transported into the cell by a bicarbonate transporter or be converted to freely diffusible CO 2 by extracellular carbonic anhydrases. Cytosolic carbonic anhydrases can produce HCO 3 − either for transport by a bicarbonate transporter into the chloroplast or for use in C 4 -like carbon-concentrating mechanisms. Chloroplastic carbonic anhydrases produces CO 2 in the vicinity of Rubisco from actively transported HCO 3 − . We were able to identify all components necessary for inorganic carbon assimilation, including putatively targeted extracellular, mitochondrial, chloroplast, and cytosolic carbonic anhydrases and bicarbonate transporters localized in the plasma membrane and in the chloroplast ( Supplementary Table S8 ). The total number of carbonic anhydrases found in N. gaditana is fewer then that found in P. tricornutum or E. siliculosus . The use of a carbonic anhydrase-type carbon-concentrating mechanism is in part supported by previous studies by Huertas and Lubian that suggested the presence of an active uptake of bicarbonate and at least intracellular carbonic anhydrases [45] , [46] , [47] . C 4 -like carbon-concentrating mechanisms have been suggested for other photosynthetic stramenopiles, including E. siliculosus , Thalassiosira weissflogii and P. tricornutum [36] , [48] , [49] . Typical C 4 metabolism relies on spatial separation between the sequestration of CO 2 into C 4 acids and the release of CO 2 from C 4 acids to Rubisco, either by differentiated cell types or the presence of specialized organelles. Single-cell C 4 -like mechanisms have recently been described in land plants, such as Bienertia sinuspersici , Bienertia cycloptera and Borszowia aralocaspia [50] , [51] , but an actual mechanism for a C 4 -like metabolism in single-cell alga has not been fully characterized. We were able to identify the genes needed for both C 3 -and C 4 -type carbon assimilation ( Supplementary Table S9 ). 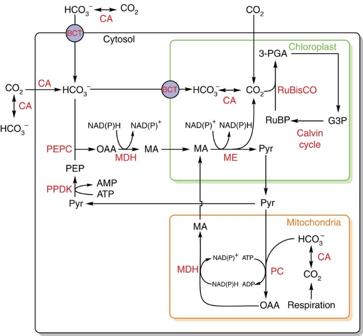Figure 6: Carbon-concentrating mechanisms. Proposed mechanisms in which inorganic carbon is assimilated byN. gaditanaand the proposed C4-like metabolism based on predicted protein localizations. Metabolites (black): G3P, glyceraldehyde 3-phosphate; MA, malic acid; OAA, oxaloacetate; PEP, phosphoenolpyruvate; 3-PGA, 3-phosphoglycerate; Pyr, pyruvate; RuBP, ribulose-1,5-bisphosphate; Enzymes (red): BCT, bicarbonate transporter; CA, carbonic anhydrase; MDH, malate dehydrogenase; ME, malic enzyme; PC, pyruvate carboxylase; PEPC, phosphoenolpyruvate carboxylase; PPDK, pyruvate, phosphate dikinase; RuBisCO, Ribulose-1,5-bisphosphate carboxylase oxygenase. TargetP [52] and HECTAR [53] were used to establish the targeting of these proteins, and a possible model for carbon-concentrating mechanisms is shown in Figure 6 . We describe two potential single cell C 4 -like carbon-concentrating mechanisms that entail production of malate in the cytosol and in the mitochondria. Both of these mechanisms rely on a chloroplast malic enzyme for release of CO 2 within the chloroplast and a malate/pyruvate shuttle that permits malate into, and pyruvate out of, the chloroplast. A similar mitochondrial-based C 4 -like mechanism has recently been described in Bienertia cycloptera [51] . Figure 6: Carbon-concentrating mechanisms. Proposed mechanisms in which inorganic carbon is assimilated by N. gaditana and the proposed C 4 -like metabolism based on predicted protein localizations. Metabolites (black): G3P, glyceraldehyde 3-phosphate; MA, malic acid; OAA, oxaloacetate; PEP, phosphoenolpyruvate; 3-PGA, 3-phosphoglycerate; Pyr, pyruvate; RuBP, ribulose-1,5-bisphosphate; Enzymes (red): BCT, bicarbonate transporter; CA, carbonic anhydrase; MDH, malate dehydrogenase; ME, malic enzyme; PC, pyruvate carboxylase; PEPC, phosphoenolpyruvate carboxylase; PPDK, pyruvate, phosphate dikinase; RuBisCO, Ribulose-1,5-bisphosphate carboxylase oxygenase. Full size image Several potential carbon-concentrating mechanisms exist in N. gaditana that may provide flexibility in carbon assimilation under a variety of environmental conditions. Further studies are needed to biochemically verify the use of these proposed carbon-concentrating mechanisms in N. gaditana . Because of the high biomass accumulation rates of N. gaditana , we also characterized genes involved in nitrogen assimilation ( Supplementary Note 4) . In addition, we also characterized genes involved in meiosis ( Supplementary Note 5) . Genetic transformation of N. gaditana using electroporation Transformation protocols for common laboratory model algae, such as C. reinhardtii and P. tricornutum have been available for more than a decade [16] , [17] , [18] , [54] , but relatively low biomass production rates in most of these strains have kept them from becoming industrially relevant. There have been reports of successful genetic transformation of Nannochloropsis oculata [55] , [56] . However, 99% of the transformants lost the transgene after 1.5 months of cultivation, indicating that the majority of the transformants had not truly incorporated the transgene into the genome. These earlier attempts, at transformation of N. oculata , relied on the use of foreign promoters, from P. tricornutum , C. reinhardtii or viral promoters and did not utilize antibiotic selection. Here we show, for the first time, the successful transformation of N. gaditana . Transformation efficiency was greatly improved by the use of endogenous promoters, identified through preliminary sequencing of the N. gaditana genome, to drive the expression of a bleomycin resistance gene. In addition, previously described protocols for the transformation of N. oculata involve the use of various enzyme mixes for creation of protoplasts before transformation [55] , [56] , whereas our protocol simply relies on the use of electroporation at high field strength. We selected three promoters for use in our transformations, which included the promoters from the genes encoding β-tubulin (TUB, Nga00092), heat shock protein 70 (HSP, Nga07210) and the ubiquitin extension protein (UEP, Nga02115.1). The efficiency of the transformations was strongly affected by the promoter used ( Table 2 ) and the most efficient transformation was achieved using the TUB promoter that resulted in an efficiency of 12.5×10 −6 . This was achieved using a very high 12,000 V cm −1 field strength during the electroporation. Use of lower field strength (10,500 V cm −1 ) resulted in fivefold lower transformation efficiency (60×10 −6 ). Interestingly, the transformation efficiency using the chosen promoters approximately corresponds with the RNAseq quantification values for these genes ( Table 2 ). We also attempted using the fucoxanthin-binding protein B (FcpB) promoter from P. tricornutum without success. The highest efficiency achieved, (12.5×10 −6 ) is comparable to the efficiency (10×10 −6 ) observed with transformations of P. tricornutum [54] . While this manuscript was in review, a report of stable transformation in Nannochloropsis W2J3B using similar electroporation parameters was published by Kilian et al . [26] Table 2 The efficiency of transformation is affected by voltage field strength and the strength of the native promoter used for expression. Full size table Confirmation of successful N. gaditana transformation was done after 4–5 months of growth with antibiotic selection. Genomic PCR confirmed the presence of the transgene in selected colonies, and Southern blot analysis confirmed successful incorporation of the transgene into the nuclear genomes of the mutant colonies ( Supplementary Fig. S7 ). The Southern blots also indicated that multiple insertions of the transgene occurred in some cases, and that integration into the genome with the construct used is random. Our results demonstrate a straightforward approach to the genetic modification of this oleaginous alga, and we anticipate that the ability to further engineer N. gaditana will allow this organism to emerge as an important model species for algal biofuel production. Here we present the annotated draft genome and a method for genetic transformation of a biofuel relevant alga, the eustigmatophyte N. gaditana . Photosynthetic algae have long been considered a possible renewable feedstock for biofuel production and have recently experienced intense interest owing to diminishing petroleum reserves and increasing atmospheric levels of CO 2 . One of the main challenges has been the lack of a genetically tractable model alga capable of industrial biofuels production. The availability of such an alga could eventually permit the sort of comprehensive systems-biology approaches that have been applied towards the development of highly productive strains of industrial bacteria. The characterization of the genome of N. gaditana and the identification of the genes and pathways that are involved in lipid production in this alga, in combination with the establishment of a method for genetic transformation, allows for further analysis of potential bottle necks in the TAG biosynthesis pathway and the discovery of suitable targets for gene overexpression and/or knockout. Several of the genes involved in TAG assembly, including PAP (Nga21116) and PDAT (Nga02737), have only one homologue and represent obvious targets for either overexpression for potential increased TAG production, or knockout for studying the physiological effects of attenuated TAG assembly. Several other identified gene families, such as TAG lipases (Nga30958, Nga30749) and acyl-CoA oxidases (Nga03053, Nga04370.1, Nga30819), as well as genes involved in gluconeogenesis are also interesting targets for gene knockout or knockdown for the purpose of increasing lipid production. In addition, both the carbonic anhydrases (Nga01240, Nga01717, Nga03728, Nga30848, Nga10007, Nga21222) and the putative bicarbonate transporters (Nga00165.01, Nga06584) are excellent targets for gene overexpression for improved carbon assimilation. The continued development of N. gaditana into a model for oleaginous algal biofuel production is a step towards the cost competitive photoautotrophic production of biofuels. Growth of N. gaditana N. gaditana CCMP526 (National Center for Marine Algae and Microbiota) was cultivated in a defined artificial seawater medium (ASW). The ASW was prepared as follows: 15 g l −1 NaCl, 6.6 g l −1 MgSO 4 ·7H 2 O, 5.6 g l −1 MgCl 2 ·6H 2 O, 0.5 g l −1 CaCl 2 ·2H 2 O, 1.45 g l −1 KNO 3 , 0.12 g l −1 KH 2 PO 4 , 0.04 g l −1 NaHCO 3 , 0.01 g l −1 FeCl 3 ·6H 2 O, 0.035 g l −1 Na 2 -EDTA, 0.25 ml l −1 3.64 mM MnCl 2 ·4H 2 O, and 0.5 ml l −1 trace metal mix (20 mg l −1 CoCl 2 ·6H 2 O, 12 mg l −1 Na 2 MoO 4 ·2H 2 O, 44 mg l −1 ZnSO 4 ·7H 2 O, 20 mg l −1 CuSO 4 ·5H2O, 7.8 g l −1 Na 2 -EDTA). The pH of the trace metal mix was adjusted to 7.5 and the final pH of the ASW was adjusted to 7.3. Low-density starting cultures were grown in low light (50 μmol m −2 s −1 ) without CO 2 supplementation. The light intensity was gradually increased and maximum biomass production was achieved from medium-density starting cultures (>3 g l −1 ) bubbled with 2% CO 2 /air at high light (200–2,000 μmol m −2 s −1 ). Estimation of biomass and lipid production yields Dry biomass yields were determined via filtration of algal cultures. The biomass from 5–10 ml of culture was collected by vacuum filtration using 0.7 μm glass fibre filters (Pall Corporation), which were then washed twice with 20 ml of diH 2 O before being dried overnight at 80 °C and then weighed. Total lipids were extracted and derivatized from liquid cultures as described previously [19] , [20] . Briefly, 1.0 ml of 1 M NaOH in 95% methanol was added to 0.5 ml of algal culture and then heated in tightly sealed vials at 100 °C for 2 h, which resulted in cell lysis and lipid saponification. Acid-catalysed methylation was accomplished by adding 1.5 ml 12 N HCl:MeOH, 1:16 (v/v) and incubating at 80 °C for 5 h. Fatty acid methyl esters (FAMEs) were extracted into 1.25 ml hexane through gentle inversion for 20 min. Extracts were washed with distilled water and analysed directly by GC-FID using an Agilent 7890A gas chromatograph with a DB-5ms column. FAMEs were quantified against a standard 37-component FAME mix (Sigma-Aldrich). Tridecanoic acid was also spiked into representative samples, and recovery of this internal standard converted to FAME was above 95%. We also verified that the conversion efficiency of TAG, free fatty acids and phospholipids was above 95% by converting standards into FAMEs. Several sources were used to determine comparative yields from different large-scale biofuel production platforms. For the production of lipids from N. gaditana , we extrapolated our small-scale yield values to large-scale production assuming 36 l per square metre. These values were corrected for 12 h:12 h light/dark cycles using a correction factor of 0.66, which we deducted from previous lipid production experiments using light/dark cycles. For soy, palm and jatropha lipid production, we used the values cited by Chisti et al . [28] For Chlorella sp. and Neochloris oleoabundans lipid production, we used values from Chen et al . [29] For the yields shown by the grey bars in Figure 1d , we utilized values derived from Atsumi et al . [30] These include S. elongatus isobutyraldehyde and isobutanol production values from their results during cultivation in 24 h light; ethanol production from S. elongatus ; hydrogen production from Anabaena variabilis , C. reinhardtii and Oscillatoria sp. ; and lipid production from Haematococcus pluvialis . DNA and RNA extraction for sequencing DNA was extracted from separate cultures as described previously [19] . Briefly, 10 ml of N. gaditana culture was pelleted and nucleic acid was extracted using phenol–chloroform according to the Newman protocol [57] and treated with RNase to degrade RNA. Nuclear, mitochondrial and plastid DNA were isolated in this fraction. RNA was extracted as previously described [19] from several different conditions and growth phases to increase the number of expressed genes. These conditions included, +/−nitrate, logarithmic phase, stationary phase, heat-shocked culture (2 h at 37 °C), cold-treated culture (2 h at 4 °C), 12-h dark acclimation, and +/−supplemental CO 2 . Aliquots of RNA from each condition were then pooled for conversion into cDNA and sequenced to obtain transcriptome data. The quality of the DNA and RNA used for sequencing was assessed by agarose-gel analysis and an Agilent Bioanalyzer, and satisfied all quality-control metrics. DNA and RNA sequencing To capitalize on their differing strengths, we employed both Roche (454) and Illumina sequencing. The relatively long sequencing reads produced by the Roche technologies are especially useful for resolving short repeated sequences during assembly. Further, we performed sequencing using an Illumina protocol called LIPES (Long insert paired-end sequencing), which pairs the sequencing reads at ~4 kb separation. The Roche 454 sequences were processed to trim off primer sequences. All sequencing reads were trimmed to an error probability of ~1:100 and to contain no ambiguous nucleotide identities. Reads shorter than 30 nucleotides were removed. Supplementary Table S10 shows the performance metrics for each type of sequencing method and Supplementary Figure S8 shows the read length distribution before and after trimming (There was little change in this for the Illumina sequencing reads.) To generate an assembled transcriptome and to map transcriptome reads to the genome for the most accurate possible gene models (using what is commonly called 'RNA-seq' methods), we generated Illumina sequencing on pooled samples of cDNA that had been made from polyA-selected RNA isolated from varying conditions (above). This cDNA was sequenced using the Illumina SIPES (Short insert paired-end sequencing) protocol, which pairs the sequencing reads at ~200 bp separation. Sequencing reads were trimmed as for the genomic sequencing data, except that all reads as long as 20 nts were retained. A total of 17,823,072 raw reads were determined and 17,723,662 survived the trimming, with a mean trimmed read length of 50.7 nts. If we assume a total transcriptome size of 11.8 MB with an average transcript length of 1,180 nts (estimated from the inferred gene content in version 1.1; see below), this corresponds to 76× sequencing coverage on a transcript represented at the mean level in these samples. Assembly of nuclear genome Numerous assemblies were performed using a variety of genome assembly programs with varying parameters followed by measuring and comparing their quality. We then used software, developed in-house, for merging of the results of the best of these various attempts into a single, well-reconciled assembly that capitalizes on the relative strengths of each type of assembly software while minimizing the chance of creating redundancy. After many trials, the best result was obtained by using Newbler version 2.3 (Roche) to assemble the Roche data and convey graph constructor (CGC; Convey Computer Corporation) to assemble the Illumina data followed by scaffold creation (based on paired-end reads that fall into adjacent contigs) using Velvet version 1.0.19 (refs 58 , 59 ). To perform the merging step, all contig/scaffold sequences from the Newbler and Velvet assemblies were first aligned all-by-all using BLASTn. Aligned pairs with a minimum reported BLAST expect value ( E -value) of 1E-7 were then screened by requiring a minimum overlapping length of 40 bp and minimum identity score of 95. The identity score was calculated as the sum of +1 for base matches, −2 penalty for mismatches, and −1 penalty for insertions or deletions (indels). As homopolymer errors are common issues for reads generated by the Roche platform, a lower indel penalty was used. A graph was then built with contigs as nodes and their pairings as edges, then continuously overlapping contigs were constructed in a greedy fashion, that is, the longest path wins in the case of conflict. In the case of conflict where one path is not significantly longer than the other (that is, differing in length by <40 nt), neither path was created. To reduce homopolymer errors from merged sequences, the consensus used the portion of the overlap taken from only the Illumina sequencing reads. We noticed that some of the scaffolds from the first assembly were likely to be bacterial. We also found that some of these scaffolds had been created from only the Illumina sequencing reads with few or no aligning Roche reads. Considering this, and suspecting that there had been some bacterial contamination specifically in the DNA preparation used for Illumina sequencing, we conducted a systematic search based on sequence matching to either bacterial or stramenopile genomic sequences and careful manual examination. This identified 363 scaffolds that contain a total of 7 Mb that were concluded to be bacterial, which were then removed along with the five scaffolds that constituted the mitochondrial and plastid genomes, leaving 2,087 scaffolds in what we designated assembly version 1.1. To estimate genome size, we subtracted duplicated regions with 100% homology from the 2,087 scaffolds. Following these corrections we assume a genome size of ~29 Mb. It takes 257 scaffolds from the assembly to contain half of the total scaffold size (the N50 statistic), and the length of the 257th longest scaffold is 37,693 nts (the L50 statistic). There are 35 scaffolds longer than 100 kb, a total of 561 longer than 20 kb, and a total of 1,447 that are longer than 2 kb. Supplementary Figure S9 shows the distribution of the paired-end separation distance for the Illumina LIPES pairs. Additional methods are found in the Supplementary Information . Accession codes: This Whole Genome Shotgun project has been deposited at DDBJ/EMBL/GenBank under the accession AGNI00000000 . The version described in this paper is the first version, AGNI01000000 . The data can also be freely accessed through the project's website, http://Nannochloropsis.genomeprojectsolutions-databases.com/ . How to cite this article: Radakovits, R. et al . Draft genome sequence and genetic transformation of the oleaginous alga Nannochloropis gaditana . Nat. Commun. 3:686 doi: 10.1038/ncomms1688 (2012).